Hydrogen bond-promoted metallic state in a purely organic single-component conductor under pressure Purely organic materials are generally insulating. Some charge-carrier generation, however, can provide them with electrical conductivity. In multi-component organic systems, carrier generation by intermolecular charge transfer has given many molecular metals. By contrast, in purely organic single-component systems, metallic states have rarely been realized although some neutral-radical semiconductors have been reported. Here we uncover a new type of purely organic single-component molecular conductor by utilizing strong hydrogen-bonding interactions between tetrathiafulvalene-based electron-donor molecules. These conductors are composed of highly symmetric molecular units constructed by the strong intra-unit hydrogen bond. Moreover, we demonstrate that, in this system, charge carriers are produced by the partial oxidation of the donor molecules and delocalized through the formation of the symmetric intra-unit hydrogen bonds. As a result, our conductors show the highest room-temperature electrical conductivity and the metallic state under the lowest physical pressure among the purely organic single-component systems, to our knowledge. Realization of purely organic single-component molecular metals has been one of the long-standing open problems in chemistry, physics and materials science. As is well known, purely organic materials are normally insulating. This is ascribable to two reasons in a band picture; (1) a valence band in organic solids is completely filled with electrons and (2) a sizable energy gap exists between the valence and conduction bands. From a molecular-level perspective, they correspond to (1) the closed-shell electron configuration of the HOMO (highest occupied molecular orbital) and (2) the large excitation energy from HOMO to LUMO (lowest unoccupied molecular orbital), together with the small intermolecular overlap of HOMOs, respectively. Then, simple ideas to produce molecular conductors are (i) to remove (add) electrons partly from HOMO (to LUMO), and (ii) to reduce the HOMO–LUMO energy gap and enhance the intermolecular orbital overlap. On the basis of the latter (ii), the nickel complex, [Ni(tmdt) 2 ] (tmdt, trimethylenetetrathiafulvalene dithiolate), has been synthesized as the first single-component molecular metal. In this material, conductive π electrons delocalize over the tetrathiafulvalene (TTF)-type large ligand skeleton, and as a result, the HOMO–LUMO gap is made smaller [1] . Subsequently, such single-component molecular conductors composed of metal complexes have been intensively developed [2] , [3] , [4] , [5] , [6] , [7] . On the other hand, the former idea (i) has given rise to the first purely organic conductor, the perylene-bromine complex [8] , followed by an enormous number of charge-transfer complexes, such as TTF-TCNQ (tetrathiafulvalene-tetracyanoquinodimethane) and BEDT-TTF (bis(ethylenedithio)tetrathiafulvalene) complexes [9] , [10] , [11] , [12] , [13] , [14] , [15] , [16] , [17] . The charge-transfer complexes are prepared by a partial electron transfer from π electron donors (for example, TTF) to acceptors (for example, TCNQ), and thus composed of two or more species in principle. The partially vacant requirement for HOMO is fulfilled not only by the charge-transfer complexes, but also by neutral-radical systems, forming the singly occupied molecular orbital (SOMO) [18] . In general, the neutral-radical system falls into the Mott insulating states, due to the intrinsic half-filled nature of the valence band consisting of the SOMO. Nevertheless, the relatively high electrical conductivity at room-temperature, σ n ~10 −6 –10 −1 S cm −1 , has been observed in several types of neutral-radical-based single-component molecular conductors [19] , [20] , [21] , [22] , [23] , [24] , [25] , [26] , [27] , [28] , [29] , [30] , [31] , [32] . So far, among the purely organic single-component systems, the metallic behaviour has been exclusively achieved under high physical pressure for some neutral-radical conductors [32] , [33] . In this paper, we unveil a new type of purely organic single-component molecular conductors based on a catechol-fused ethylenedithiotetrathiafulvalene, H 2 Cat-EDT-TTF, and its diselena analogue, H 2 Cat-EDT-ST ( Fig. 1a ), which are designed and synthesized by us [34] . These conductors are unprecedented single-component systems composed of the molecular units, H 3 (Cat-EDT-TTF) 2 and H 3 (Cat-EDT-ST) 2 , with a highly symmetric intra-unit hydrogen bonds ( Fig. 1b ). Their electrical conductivity at room-temperature, σ n ~3.5–19 S cm −1 , is significantly higher than that for the previously reported purely organic single-component systems (see above). Under physical pressure above greater than 1.3 GPa, moreover, the metallic behaviour appears in the temperature dependence of the electrical resistivity. The higher electrical conductivity observed in our systems is attributed to the hydrogen bond-promoted delocalization of charge carriers, which are generated through the partial oxidation of the H 2 Cat-EDT-TTF and H 2 Cat-EDT-ST molecules. 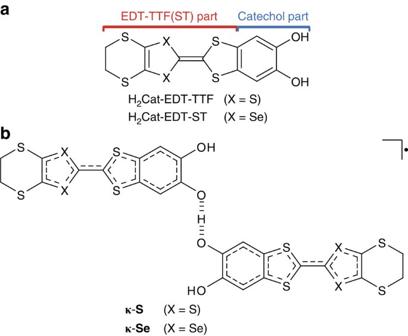Figure 1: Chemical structures of the molecules in text. (a) H2Cat-EDT-TTF and H2Cat-EDT-ST molecules. (b) A hydrogen-bonded molecular unit,κ-Sandκ-Se. Figure 1: Chemical structures of the molecules in text. ( a ) H 2 Cat-EDT-TTF and H 2 Cat-EDT-ST molecules. ( b ) A hydrogen-bonded molecular unit, κ-S and κ-Se . Full size image Crystal and electronic structures A new type of purely organic single-component molecular conductors, κ-H 3 (Cat-EDT-TTF) 2 and κ-H 3 (Cat-EDT-ST) 2 , hereinafter described as κ-S and κ-Se , respectively, were obtained as black plate-like crystals by electrochemical oxidation of the corresponding donor molecules, H 2 Cat-EDT-TTF and H 2 Cat-EDT-ST ( Fig. 1a ) [34] , in the presence of the base, 2,2′-bipyridine (see methods ). We emphasize here that κ-S and κ-Se are isostructural with each other, as revealed by the X-ray diffraction measurements using their high-quality single crystals. Thus, the structural features for κ-S described below are essentially the same as those for κ-Se . First, we focus on the distinctive building block in a unit cell, the minimal molecular unit , displayed in Figs 1b and 2 . The minimal molecular unit, the H 3 (Cat-EDT-TTF) 2 composition, is established by the formation of an intra-unit hydrogen bond, O…H…O, between the catechol moieties of the donor molecules, where the one hydroxyl proton is deprotonated. The oxygen–oxygen distance in the hydrogen bond, d oo , is 2.486(5) Å and 2.509(8) Å at room-temperature, and 2.453(5) Å and 2.443(8) Å at 50 K and 30 K for κ-S and κ-Se , respectively, which are much shorter than the length of the normal O–H…O type hydrogen bond, d oo ~2.7–3.0 Å [35] , [36] (refs35,36). These short distances are an evidence of the considerably high-bonding energy of the hydrogen bonds for both κ-S and κ-Se . Because of this strong hydrogen bonding nature, the bonded hydrogen atom is nearly located at the centre between two oxygen atoms, in contrast to the asymmetric hydrogen distribution in the normal hydrogen bonds. The bilateral Cat-EDT-TTF parts connected by the hydrogen bond are related by twofold rotational symmetry with respect to the central hydrogen atom, namely, crystallographically equivalent with each other. The density functional theory (DFT) calculations of this minimal molecular unit at the ROB3LYP/6-31G(d) level suggest that the HOMO of the minimal unit is spread not only on the TTF part, but also on the oxygen atoms in the catechol part, as shown in Fig. 2b . Therefore, the π electrons are widely delocalized over the whole minimal molecular unit. 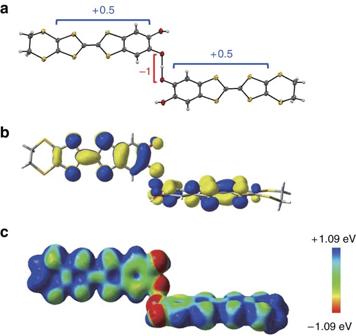Figure 2: X-ray crystal structure and computation results showing the hydrogen-bonding in κ-S. (a) The minimal molecular unit in a unit cell,κ-Scomposition. The white spheres, grey, red and yellow ellipsoids represent the hydrogen, carbon, oxygen and sulphur atoms, respectively. All the ellipsoids are drawn at the 50% probability level. (b) The HOMO distribution in the minimal unit calculated at the ROB3LYP/6-31 G(d) level of theory. (c) The electrostatic potential surface of the minimal unit calculated at the UB3LYP/6-31G(d) level of theory. Figure 2: X-ray crystal structure and computation results showing the hydrogen-bonding in κ-S. ( a ) The minimal molecular unit in a unit cell, κ-S composition. The white spheres, grey, red and yellow ellipsoids represent the hydrogen, carbon, oxygen and sulphur atoms, respectively. All the ellipsoids are drawn at the 50% probability level. ( b ) The HOMO distribution in the minimal unit calculated at the ROB3LYP/6-31 G(d) level of theory. ( c ) The electrostatic potential surface of the minimal unit calculated at the UB3LYP/6-31G(d) level of theory. Full size image Next, let us discuss the charge states of the minimal molecular unit. Considering the −1 valence state of the deprotonated O…H…O hydrogen bond, we can expect the +0.5 state of a TTF part to remain neutral as the whole of the minimal unit. Experimentally, the +0.5 valence state is confirmed by the empirical bond-length analyses (see Supplementary Fig. S1 , Supplementary Table S1 , and Supplementary Methods ), meaning that the TTF part is partially oxidized in the construction process of the minimal molecular unit. The charge distribution is also evaluated by the electrostatic potential of the minimal unit obtained by the UB3LYP/6-31G(d) calculations ( Fig. 2c ). As shown in Fig. 2c , the positive charge is extensively distributed over the EDT-TTF part, while the oxygen atoms favour negative charge, associated with the [O…H…O] − state. Thus, charge carriers are generated for κ-S , probably κ-Se as well. The minimal molecular units are assembled into the purely organic single-component crystal, as shown in Fig. 3a , Supplementary Figs S2 and S3 . The order of the minimal unit looks like a periodic layered structure along the crystal a axis. In fact, a large number of charge-transfer complexes based on TTF derivatives form the layer structure, which are usually composed of conducting electron-donor layers and insulating counter-anion layers [9] , [10] , [11] , [12] , [13] , [14] , [15] , [16] , [17] . In our case, however, each Cat-EDT-TTF part connected by the hydrogen bond belongs to the neighbouring layers, as shown in the pink and blue molecular units in Fig. 3a . These two units form a dimeric structure in a layer, which is clearly seen in the cross-section view perpendicular to the molecular long axis ( Fig. 3b ). As shown in Fig. 3b , two Cat-EDT-TTF skeletons in the pink and blue molecular units come face-to-face to form the dimeric structure. Each dimer is orthogonally arranged with the zigzag pattern, which is traditionally termed as the ‘‘κ-type’’ molecular arrangement in the field of the BEDT-TTF-based molecular conductors [37] , [38] , [39] . In the present molecular arrangement, there exist the intra- and inter-dimer short atomic contacts of S…S ~3.54 and 3.45–3.56 Å (Se…S~3.59–3.64 and 3.50–3.66 Å), respectively, for κ-S ( κ-Se ), as shown in the dotted lines. All of them are shorter than the sum of the van der Waals radius of sulphur and selenium atoms, that is S…S~3.60 Å and Se…S~3.70 Å, indicating that the π molecular orbitals of the minimal unit are overlapped not only within the dimer but also between the dimers. 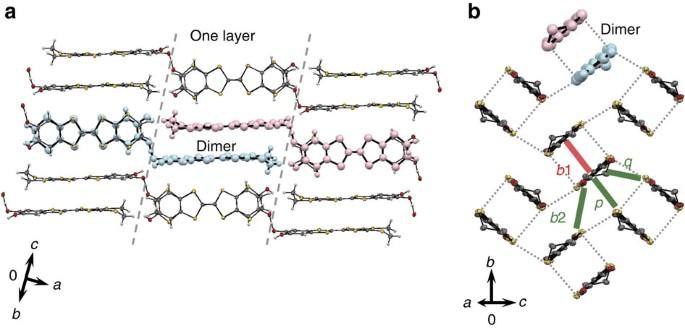Figure 3: Crystal packing structure of κ-S. (a) The arrangement of the minimal molecular unit. Two units are highlighted by the pink and light blue spheres. (b) The cross-section view perpendicular to the molecular long axis. The dimeric structure is depicted by the pink and light blue spheres, which correspond to that inFig. 3a. The transfer integralsb1,b2,pandqare 230 (318), 85.4 (140), 45.9 (63.9) and −11.7 meV (−21.4 meV) at 50 K (30 K) forκ-S(κ-Se), respectively. The grey, red and yellow ellipsoids represent the carbon, oxygen and sulphur atoms, respectively. All the ellipsoids are drawn at the 50% probability level. The short S…S atomic contacts are shown by the grey dotted line. Figure 3: Crystal packing structure of κ-S. ( a ) The arrangement of the minimal molecular unit. Two units are highlighted by the pink and light blue spheres. ( b ) The cross-section view perpendicular to the molecular long axis. The dimeric structure is depicted by the pink and light blue spheres, which correspond to that in Fig. 3a . The transfer integrals b 1, b 2, p and q are 230 (318), 85.4 (140), 45.9 (63.9) and −11.7 meV (−21.4 meV) at 50 K (30 K) for κ-S ( κ-Se ), respectively. The grey, red and yellow ellipsoids represent the carbon, oxygen and sulphur atoms, respectively. All the ellipsoids are drawn at the 50% probability level. The short S…S atomic contacts are shown by the grey dotted line. Full size image On the other hand, there exist no short intermolecular S…S or Se…S contacts along the a axis ( Fig. 3a ), meaning that the intermolecular interactions between the layers is considerably weaker than the intra- and inter-dimer interactions mentioned above. On the basis of this fact, assuming that the intermolecular interactions between the layers is negligible, we estimate the two-dimensional electronic band structure through the tight-binding approximation using the intra- and inter-dimer transfer integrals, b 1, b 2, p and q ( Fig. 3b ). They were obtained by the extended Hückel method calculations [40] , [41] , [42] . 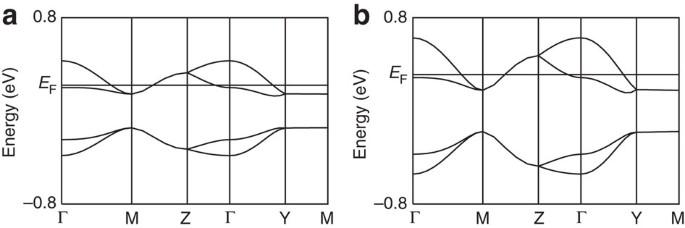Figure 4: Electronic band structure. The two-dimensional energy dispersion in the first Brillouin zone for (a) κ-H3(Cat-EDT-TTF)2and (b) κ-H3(Cat-EDT-ST)2. Figure 4a show the electronic band structure consisting of four independent HOMOs for κ-S and κ-Se , respectively. The band width for κ-Se is found to be larger than that for κ-S . This is because the introduction of the spatially extensive atomic orbital of selenium effectively enhances the intermolecular orbital overlap. Considering the +0.5 oxidized state of the TTF and ST parts in the minimal molecular unit, a quarter of the HOMO bands is occupied by holes; the hole quarter-filled band is formed. However, the large band splitting between the upper and lower bands, comparable to the band width, provides a half-filled character for the electronic bands associated with the dimer-Mott states. Figure 4: Electronic band structure. The two-dimensional energy dispersion in the first Brillouin zone for ( a ) κ-H 3 (Cat-EDT-TTF) 2 and ( b ) κ-H 3 (Cat-EDT-ST) 2 . Full size image Electrical resistivity Temperature-dependent electrical resistivity ρ ( T ) for κ-S and κ-Se is shown in Fig. 5a . First, note that the electrical conductivity at room-temperature, σ rt =1/ ρ rt , is significantly high, ~3.5 and 19 S cm −1 for κ-S and κ-Se , respectively. These values are one or two orders of magnitude higher than the highest reported value, σ n ~10 −1 S cm −1 , in the purely organic single-component systems, to our best knowledge [20] , [23] , [24] , [26] , [27] . As temperature is decreased, the electrical resistivity of these systems exponentially increases, which is a typical semiconducting behaviour, ρ ( T ) exp(Δ/2 k B T ), and consistent with the results of the electronic band calculations. Here, Δ and k B are the semiconducting energy gap and the Boltzmann constant, respectively. The energy gap Δ/ k B , estimated by the slope of the ln ρ versus 1,000/ T plot ( Fig. 5b ), is 2400 K for κ-S and 1200 K for κ-Se , respectively. 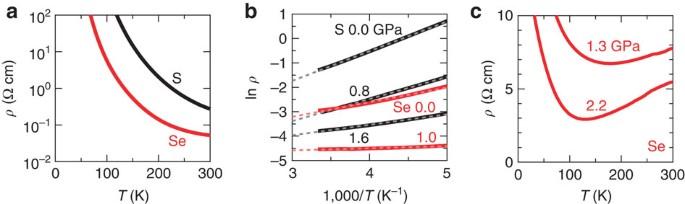Figure 5: Electrical resistivity of κ-S and κ-Se. (a) The electrical resistivity as a function of temperature at ambient pressure. The black and red plots exhibit the resistive curves forκ-Sandκ-Se, respectively. (b) lnρversus 1,000/Tplot at ambient pressure and under the physical pressure. The dashed lines show the line fitting for the lnρcurves in the temperature range of 200–300 K. (c) Temperature dependence of the electrical resistivity under the pressure of 1.3 and 2.2 GPa forκ-Se. Figure 5: Electrical resistivity of κ-S and κ-Se. ( a ) The electrical resistivity as a function of temperature at ambient pressure. The black and red plots exhibit the resistive curves for κ-S and κ-Se , respectively. ( b ) ln ρ versus 1,000/ T plot at ambient pressure and under the physical pressure. The dashed lines show the line fitting for the ln ρ curves in the temperature range of 200–300 K. ( c ) Temperature dependence of the electrical resistivity under the pressure of 1.3 and 2.2 GPa for κ-Se . Full size image The physical pressure is a good tool to change the electronic states by the modulation of the intermolecular interactions. Thus, we measured the electrical conductivity under the pressure for our purely organic single-component molecular conductors. It is obvious that the application of pressure reduces the slope of the ln ρ curve, concurrently with the enhancement of the electrical conductivity, as shown in Fig. 5b . This result is clearly an indication of the monotonic decrease of the semiconducting energy gap with increasing pressure. Up to 1.6 GPa, however, κ-S still remains semiconductive. On the other hand, we observed dramatic changes in the temperature variation in the electrical resistivity under pressure for κ-Se , as displayed in Fig. 5c . The room-temperature electrical conductivity is significantly enhanced with pressure, σ n ~180 S cm −1 at 2.2 GPa. This value is an order of magnitude higher than σ rt at ambient pressure. Under the pressure above 1.3 GPa, the electrical resistivity monotonically decreases with reducing temperature down to around 150 K, in striking contrast with the semiconducting behaviour at ambient pressure, although the resistive curve turns to increase at low temperature. Thus, the metallic states emerge with the simultaneous suppression of the semiconducting energy gap by the application of the pressure of only ~1 GPa. To our knowledge, this is the lowest metallization pressure among the purely organic single-component systems [32] , [33] , [43] , [44] . An important question is the reason why the significantly high electrical conductivity is achieved for the purely organic single-component systems κ-S and κ-Se . The hole generation by the partial oxidation of the TTF and ST parts in the minimal molecular unit resembles that in the charge-transfer complexes rather than the intrinsic half-filled electron configuration of SOMO in the neutral radicals. In the case of the normal charge-transfer complexes, the charge carriers are produced by the redox reaction between the electron donors and acceptors. In our systems, however, there exist no counter components to accept the electrons transferred from the π electron-donor molecules by oxidation. Instead, it should be noted that the [O…H…O] − hydrogen bond compensates the positive charge to remain neutral as the whole of the minimal molecular unit. At the moment, the detailed process of the formation of the minimal unit and the electrochemical crystallization is unclear. On the analogy of the formation of phosphonic-acid and amino-acid TTFs [45] , [46] , however, the process is possibly explained as follows; H 2 Cat-EDT-TTF is diacid. In the presence of bipyridine (see methods ), the monoanionic (HCat-EDT-TTF) − is generated. This anionic species oxidizes at a lower potential than H 2 Cat-EDT-TTF itself into the zwitterionic (HCat-EDT-TTF) · . Because of the adapted choice of base, both H 2 Cat-EDT-TTF and (HCat-EDT-TTF) · are then present in solution and co-crystallize, through the symmetric hydrogen bond. As a result of the formation of the highly symmetric molecular unit, the HOMO distribution is widely extended over the whole molecular unit, as shown in Fig. 2b . The widely extended π-electron molecular orbital effectively suppresses the on-site Coulomb repulsion, giving rise to the enhancement of the intermolecular carrier movement. Therefore, the construction of the molecular unit provides an itinerant character for the generated carriers. It is also important that each H 3 (Cat-EDT-TTF) 2 (H 3 (Cat-EDT-ST) 2 ) unit of κ-S ( κ-Se ) is assembled into the κ-type molecular arrangement observed in the usual BEDT-TTF-based charge-transfer complexes, leading to the relatively strong intermolecular interactions. In fact, κ-type BEDT-TTF complexes exhibit the metallic phase including superconducting states by overcoming the Mott insulating states through the control of the band width [16] , [17] . Thus, in spite of the purely organic single-component systems, κ-S and κ-Se form the partly-filled valence band, and consequently, exhibit the highest electrical conductivity among the purely organic single-component molecular conductors. In κ-Se , moreover, we found the metallic states by the application of the lowest physical pressure among the purely organic single-component systems. Most studies of the molecular conductors based on hydrogen bond-functionalized TTF derivatives have focused on the tuning of the molecular self-assembly and the HOMO/LUMO energy levels [47] , [48] . In this context, several groups have recently reported that the introduction of the hydrogen bond has another important role, that is, the generation of the charge carriers [46] , [49] . Besides the carrier generation, our system demonstrates that the symmetric hydrogen bond constructs the new type of the purely organic single-component molecular conductors which are composed of highly symmetric molecular units. Moreover, we found that the formation of the symmetric hydrogen bond promoted the intermolecular delocalization of the generated carriers, associated with the enhancement of the electrical conductivity. We believe that our new type of molecular conductors with the symmetric intra-unit hydrogen bond will realize the first purely organic single-component molecular metal at ambient pressure. A tetraselenafulvalene-type analogue, in which all the sulphur atoms in the TTF part of the present system are replaced with selenium atoms, is a promising candidate for the ambient-pressure metal, because the further enhanced intermolecular interactions are expected. The preparation of this new donor molecule, as well as its purely organic single-component conductor is currently underway in our laboratory. Sample preparation The donor molecules H 2 Cat-EDT-TTF and H 2 Cat-EDT-ST were prepared according to the literature [34] . Black plate-like single crystals of purely organic single-component conductors κ-H 3 (Cat-EDT-TTF) 2 and κ-H 3 (Cat-EDT-ST) 2 were grown by the electrochemical oxidation of the donors H 2 Cat-EDT-TTF (12 mg, 0.03 mmol) and H 2 Cat-EDT-ST (10 mg, 0.02 mmol) in a chlorobenzene/acetone solution including 2,2′-bipyridine (15 mg, 0.10 mmol and 5.7 mg, 0.04 mmol, respectively) as a base and n -Bu 4 NPF 6 (40 mg, 0.10 mmol) as a electrolyte. In the electrochemical oxidation, constant current (0.2 μA) was applied between two annealed Pt electrodes at 30 °C during 10 days. As-grown high-quality single crystals with the typical size of 150 × 50 × 10 μm 3 and 500 × 100 × 10 μm 3 were used for the X-ray diffraction and the electrical resistivity measurements, respectively. X-ray crystal structure analysis X-ray diffraction experiments were performed by using the MoK α radiation ( λ = 0.71069 Å) at Institute for Molecular Science, Japan, and the synchrotron radiation source ( λ =1.0 Å) at PF BL-8 A in High Energy Accelerator Research Organization (KEK), Japan. The diffraction data were collected on the CCD diffractometer (Rigaku) at Institute for Molecular Science and the Imaging plate system (Rigaku) at KEK ( Supplementary Table S2 ), which adopted a cold helium gas flow-type system for the low-temperature experiments. The crystal structure was solved through the direct method. Refinement was carried out by a full-matrix least-squares method (SHELXL97), in which the anisotropic temperature factors are refined for all the atoms except for the hydrogen atoms. The thermal disorder of the terminal ethylenedithio part was observed at room-temperature for both κ-S and κ-Se . Thus, the discussion about the crystal structures in the text was mainly performed by using the low-temperature diffraction data. Theoretical calculations All DFT calculations were performed with Gaussian 03, revision E.01 (ref. 50 ). The band structure calculations were performed with the extended Hückel method by using the tight-binding approximation [40] . The molecular geometry of the hydrogen-bonded minimal unit of κ-S and κ-Se was taken from the X-ray analysis data measured at 50 and 30 K, respectively. Electrical resistivity under pressure Electrical resistivity was measured by the conventional four probe ac method on the Physical Properties Measurement System (Quantum Design). The annealed Au wires ( φ = 15 μm) were attached on the single crystal by the carbon paste. The physical pressure was applied through the Ni-Cr-Al piston-cylinder-type pressure cell enclosing the sample and the pressure medium, Daphne 7373. The applied pressure was estimated by the pressure variation in the superconducting transition temperature of lead: d T c /d P =−0.365 K GPa −1 ( [51] ). Accession codes : The X-ray crystallographic coordinates for structures reported in this article have been deposited in the Cambridge Crystallographic Data Centre (CCDC), under deposition numbers CCDC 894470–894473. These data can be obtained free of charge from The Cambridge Crystallographic Data Centre via http://www.ccdc.cam.ac.uk/datarequest/cif How to cite this article: Isono, T. et al . Hydrogen bond-promoted metallic state in a purely organic single-component conductor under pressure. Nat. Commun. 4:1344 doi: 10.1038/ncomms2352 (2013).